VapC20 ofMycobacterium tuberculosiscleaves the Sarcin–Ricin loop of 23S rRNA The highly persistent and often lethal human pathogen, Mycobacterium tuberculosis contains at least 88 toxin–antitoxin genes. More than half of these encode VapC PIN domain endoribonucleases that inhibit cell growth by unknown mechanisms. Here we show that VapC20 of M. tuberculosis inhibits translation by cleavage of the Sarcin–Ricin loop (SRL) of 23S ribosomal RNA at the same position where Sarcin and other eukaryotic ribotoxins cleave. Toxin-inhibited cells can be rescued by the expression of the antitoxin, thereby raising the possibility that vapC20 contributes to the extreme persistence exhibited by M. tuberculosis . VapC20 cleavage is inhibited by mutations in the SRL that flank the cleavage site but not by changes elsewhere in the loop. Disruption of the SRL stem abolishes cleavage; however, further mutations that restore the SRL stem structure restore cleavage, revealing that the structure rather than the exact sequence of the SRL is important for this activity. M ycobacterium tuberculosis , the deadliest human pathogenic bacterium, possesses the ability to persist within its host for decades [1] . Many other pathogenic bacteria have the ability to generate chronic or relapsing infections, and the problem of bacterial persistence is of general importance [2] , [3] , [4] . The molecular mechanisms underlying bacterial persistence have been difficult to analyse, not least because of the low frequencies of persisters in growing bacterial cultures (typically 10 −4 –10 −6 of the cell population). However, persistence of the model organism Escherichia coli depends on induction of type II toxin–antitoxin (TA) activity by (p)ppGpp, the concentration of which varies stochastically in growing bacteria [5] , [6] . (p)ppGpp stimulates the accumulation of polyphosphate by inhibiting exopolyphosphatase, the major polyphosphate-degrading enzyme of E. coli . In turn, polyphosphate activates Lon protease to degrade antitoxins, thereby leading to activation of the toxins. The TA gene-encoded toxins of E. coli inhibit translation and cell growth, and thereby induce multidrug tolerance and persistence. Because of these observations, it has becomes important to understand the biology and targets of prokaryotic type II TA modules. Almost all type II TA genes code for two proteins, a toxin that inhibits cell growth and an antitoxin that counteracts the toxin by direct protein–protein interaction. The TA operons are usually autoregulated by the TA complex that binds cooperatively to operators in the promoter region. Even though the antitoxin is labile, its rate of synthesis is sufficiently high to generate a steady-state level of antitoxin that is higher than that of the toxin in exponentially growing cells. However, in starved or otherwise slow-growing cells, protease-mediated degradation of antitoxin may lead to toxin activation and inhibition of translation [7] . A wide variety of prokaryotic TA genes have been identified and some organisms carry highly expanded repertoires of them within their chromosomes [8] . M. tuberculosis has at least 88 type II TA loci that may contribute to the virulence and extreme persistence of the organism [9] . Consistent with this hypothesis, ten different TAs were activated in persister cell populations of M. tuberculosis [10] . Moreover, ectopic expression of type II toxins in M. tuberculosis induces a dormant, drug-tolerant state [11] . Finally, in a proteomics study, the protein levels of 14 TA-encoded toxins of M. tuberculosis were observed to increase in response to nutrient limitation, indicating a role of these systems also in stress response and growth adaptation [12] . On the basis of toxin gene similarities, type II TA loci have been divided into gene families of independent evolutionary origin [8] . The most abundant TA gene family, vapBC (virulence associated protein), is common in both bacteria and archaea [8] . Remarkably, some organisms, such as M. tuberculosis H37Rv, have vastly expanded repertoires of TA genes. This organism has 88 known type II TA modules, of which 45 are vapBC loci [8] , [9] . VapC toxins are PIN ( pi lT amino-terminal) monodomain endoribonucleases containing three or four acidic residues that coordinate Mg 2+ ion(s) in the active site [13] . In eukaryotes, PIN domains are present in multidomain proteins involved in RNA metabolism, RNA quality control and rRNA maturation [14] . For example, Nob1 contains a PIN domain that cleaves rRNA site specifically during ribosome biogenesis [15] , [16] , [17] , [18] . The molecular targets of prokaryotic VapC PIN domain nucleases are in most cases unknown; however, we showed recently that enteric VapCs cleaved initiator transfer RNA site specifically in the anticodon loop and thereby efficiently inhibited global translation [19] . Interestingly, many other VapC toxins that were analysed also inhibited cell growth, but their specific cellular targets were not identified. Three different research groups showed that VapC20 (Rv2549c) of M. tuberculosis H37Rv inhibited the growth of E. coli , M. smegmatis and M. tuberculosis [20] , [21] , [22] . However, the mechanism behind the observed growth inhibition remained unknown. Here we show that VapC20 prevents bacterial cell growth by inhibiting global translation through endonucleolytic cleavage of the tetraloop of Helix 95 of 23S rRNA. This structure, also known as the Sarcin–Ricin loop (SRL), is universally conserved in all domains of life and is the target of the deadly eukaryotic toxins, α-Sarcin and Ricin. Remarkably, VapC20 and Sarcin cleave the SRL loop at exactly the same position. VapC20 inhibits cell growth and translation VapC20 of M. tuberculosis is encoded by the bicistronic vapBC20 operon ( Fig. 1a ). To study the effect of expression of VapC20 in E. coli , we modified the vapC20 gene to optimize translation initiation and inserted it downstream of a plasmid-encoded arabinose-inducible promoter. As expected, induction of vapC20 results in growth inhibition and a dramatic, 10,000-fold reduction in the number of colony-forming units (CFUs) ( Fig. 1b ). Concomitantly, the global rate-of-translation is severely reduced ( Fig. 1c ). Analogous experiments show that transcription and replication, respectively, are not affected by induction of vapC20 (see Supplementary Fig. S1A,B ). 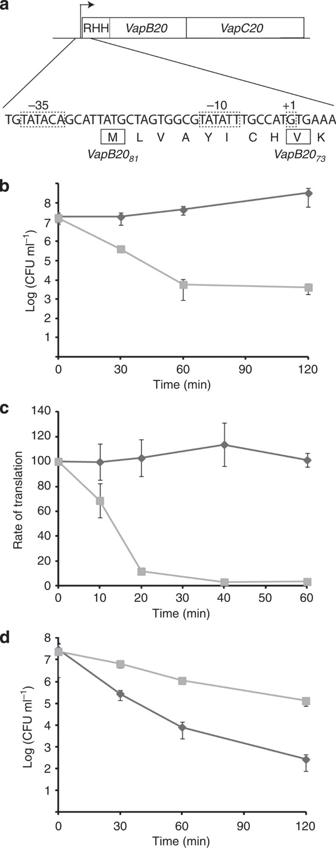Figure 1: VapC20 inhibits cell growth and translation. (a) Schematic representation of thevapBC20locus ofM. tuberculosisH37rv. Two versions ofvapB20are shown, one as originally annotated (vapB2081) and the other as re-annotated here (vapB2073). The transcriptional start site of thevapBC20operon was obtained by deep RNA sequencing by D. Young’s (personal communication) group at the National Institute for Medical Research, London, UK; corresponding –10 and –35 promoter sequences are indicated by dashed boxes and RHH indicates part ofvapB20encoding Ribbon–Helix–Helix DNA-binding domain (b) Effect of ectopic expression of VapC20 on viable cell counts (CFU). Cells of MG1655 containing pBAD33 control (diamonds) or pKW332549c (PBAD::SDop::vapC20) (squares) were grown exponentially in LB medium at 37 °C. At time zero,vapC20was induced by 0.2% arabinose. Cell samples were removed at time points indicated, diluted and plated on solid medium with glucose. The data reflect three independent experiments including s.d. (c) VapC20 inhibits translation. Two cultures ofE. coliK-12 cells containing plasmid pKW332549c (PBAD::SDop::vapC20) were grown exponentially in M9 minimal medium at 37 °C. At time zero, one culture was induced with 0.2% arabinose (squares), whereas one was left uninduced (diamonds). Cell samples were collected at the time points indicated and pulsed for 1 min with radiolabelled35S-methionine. Data are shown as a rates-of-translation by averaging three independent experiments with resulting s.d.; time zero rates-of-translation were set to 100%. The values were adjusted for differences in cell densities. (d) Resuscitation of VapC20-inhibited cells. Cells of MG1655 containing pKW332549c (PBAD::SDop::vapC20) and pKW222550copLL (PA1/O3/O4::SDop::vapB2073) were grown exponentially in LB medium at 37 °C. At time zero,vapC20was induced by 0.2% arabinose. Cell samples were removed at time points indicated, diluted and plated on solid medium with (squares) or without (diamonds) 2 mM IPTG. The curves shown were averages of three independent experiments with resulting s.d. Figure 1: VapC20 inhibits cell growth and translation. ( a ) Schematic representation of the vapBC20 locus of M. tuberculosis H37rv. Two versions of vapB20 are shown, one as originally annotated ( vapB20 81 ) and the other as re-annotated here ( vapB20 73 ). The transcriptional start site of the vapBC20 operon was obtained by deep RNA sequencing by D. Young’s (personal communication) group at the National Institute for Medical Research, London, UK; corresponding –10 and –35 promoter sequences are indicated by dashed boxes and RHH indicates part of vapB20 encoding Ribbon–Helix–Helix DNA-binding domain ( b ) Effect of ectopic expression of VapC20 on viable cell counts (CFU). Cells of MG1655 containing pBAD33 control (diamonds) or pKW332549c (P BAD ::SD op :: vapC20 ) (squares) were grown exponentially in LB medium at 37 °C. At time zero, vapC20 was induced by 0.2% arabinose. Cell samples were removed at time points indicated, diluted and plated on solid medium with glucose. The data reflect three independent experiments including s.d. ( c ) VapC20 inhibits translation. Two cultures of E. coli K-12 cells containing plasmid pKW332549c (P BAD ::SD op :: vapC20 ) were grown exponentially in M9 minimal medium at 37 °C. At time zero, one culture was induced with 0.2% arabinose (squares), whereas one was left uninduced (diamonds). Cell samples were collected at the time points indicated and pulsed for 1 min with radiolabelled 35 S-methionine. Data are shown as a rates-of-translation by averaging three independent experiments with resulting s.d. ; time zero rates-of-translation were set to 100%. The values were adjusted for differences in cell densities. ( d ) Resuscitation of VapC20-inhibited cells. Cells of MG1655 containing pKW332549c (P BAD ::SD op :: vapC20 ) and pKW222550copLL (P A1/O3/O4 ::SD op :: vapB20 73 ) were grown exponentially in LB medium at 37 °C. At time zero, vapC20 was induced by 0.2% arabinose. Cell samples were removed at time points indicated, diluted and plated on solid medium with (squares) or without (diamonds) 2 mM IPTG. The curves shown were averages of three independent experiments with resulting s.d. Full size image To assess the effect of expression of VapC20 in a mycobacterial strain, we inserted the vapC20 gene into a shuttle vector downstream of an inducible promoter and transferred the plasmid to M. smegmatis . As with E. coli , induction of vapC20 severely inhibits the growth of this organism (see Supplementary Fig. S1C ). In summary, our results show that VapC20 specifically inhibits growth and translation. Induction of vapB20 can resuscitate VapC20-inhibited cells The VapB20 antitoxin encoded by vapB20 (Rv2550c) is predicted to be 81 amino acids long. However, unpublished RNAseq data indicate that the vapBC20 operon messenger RNA is leaderless and that translation starts at the internal GTG valine codon at +9 of the annotated vapB20 gene ( Fig. 1a , D. Young, personal communication). In support of this annotation, the transcription start site generating the leaderless mRNA is preceded by suitable –10 (TATATT) and –35 (TATACA) promoter sequences ( Fig. 1a ). Together, these observations suggest that VapB20 is instead 73 amino acids with the Ribbon–Helix–Helix DNA-binding motif located at its very N terminus ( Fig. 1a ). To test this, we initially placed E. coli codon-optimized versions of both the full-length gene, vapB20 81 , and the shorter version predicted to be encoded by the leaderless mRNA ( vapB20 73 ), downstream of an isopropyl-β- D -thiogalactoside (IPTG)-inducible promoter. We observe that both versions counteract VapC20 (see Supplementary Fig. S1D ). We conclude that vapB20 73 encodes a functional VapB20 antitoxin that is likely to be the native antitoxin produced by M. tuberculosis . In the following, VapB20 denotes the 73 aa antitoxin and vapB20 the corresponding gene. Toxins encoded by type II TA loci commonly induce stasis from which the cells can be resuscitated [23] , [24] , [25] . It has previously been shown that coexpression of VapB20 81 can counteract VapC20 toxicity when encoded by a plasmid in E. coli or M. smegmatis , or by the chromosomal vapBC20 locus in M. tuberculosis [21] , [22] . Therefore, we decided to measure whether induction of vapB20 can revive cells that had previously been inhibited by induction of vapC20 . To this end, we constructed a strain containing vapC20 and vapB20 with optimized translation initiation signals under arabinose and IPTG control, respectively (P BAD ::SD opt :: vapC20 and P A1/O3/O4 :: SD opt :: vapB20 ). As shown above, induction of only vapC20 results in a dramatic reduction of the number of CFU ( Fig. 1d ). However, subsequent induction of vapB20 (by plating the cells on solid medium with IPTG) significantly reduces the toxicity of vapC20 . We conclude that the expression of VapB20 allows a significant part of cells that have been inhibited by ectopic overproduction of VapC20 to regrow. VapC20 cleaves 23S rRNA First, we tested whether the VapC20-mediated inhibition of translation is due to cleavage of tRNA as in the cases of enteric VapCs [19] . However, induction of vapC20 does not change the abundance of any of the tested tRNA species, including tRNA fMet , tRNA Thr1 , tRNA His , tRNA Phe , tRNA Arg2 , tRNA Tyr and tRNA Val (see Supplementary Fig. S2A ). To further pursue the idea of a possible tRNAse activity of VapC20, we compare total RNA purified from E. coli cells expressing VapC of plasmid pMYSH6000 from Shigella flexneri and VapC20 of M. tuberculosis ( Fig. 2a ). A cleavage product, corresponding to the expected tRNA fragment is detected after induction of vapC of S. flexneri , whereas no such fragment is seen after induction of vapC20 . Instead, an ~250 nt RNA fragment accumulates after vapC20 induction. A similar RNA fragment is observed when VapC20 is expressed in M. smegmatis (see Supplementary Fig. S3A ). Northern blotting analysis reveals that the RNA fragment is a cleavage product of the 3′-end of 23S rRNA (see Supplementary Fig. S2B ). No cleavage of 16S rRNA is detected (see Supplementary Fig. S2C ). A 23S rRNA-derived cleavage fragment is also observed when VapC20 is expressed in M. smegmatis (see Supplementary Fig. S3B ). Neither induction of vapC MYSH nor inhibition of translation by chloramphenicol (Cm) change the observed 23S rRNA cleavage pattern (see Supplementary Fig. S2B ). Finally, change of a conserved active site residue (D5A) of VapC20 abolishes the formation of the 23S rRNA fragment showing that the rRNA fragment is the direct result of the enzymatic activity of VapC20 (see Supplementary Fig. S2D ). 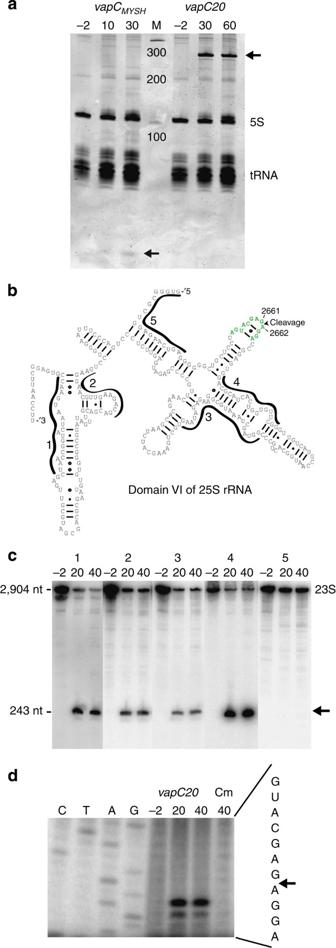Figure 2: VapC20 cleaves the SRL loop of 23S rRNA. (a) Analysis of total RNA fromE. coli. MG1655/pKW82 (PBAD::vapCMYSH; left panel) and MG1655/pKW332549c (PBAD::SDop::vapC20; right panel) were grown exponentially in LB medium and transcription induced at time zero by the addition of arabinose (0.2%). Cell samples were collected at the time points indicated (min). Total RNA extracted from the samples were separated on a 4.5% denaturing polyacrylamide gel and visualized by ethidium bromide staining. M denotes an RNA size marker. VapC cleavage products are indicated with arrows. (b) The position of the probes used incare indicated in the secondary structure of domain VI of 23S rRNA. The universally conserved nucleotides in the SRL loop of Helix 95 are indicated in green and the VapC20 cleavage site by an arrow. (c) Mapping of the cleavage site by northern blot analysis. Cells of MG1655/ pKW332549c (PBAD::SDop::vapC20) were grown exponentially in LB medium. At time zero, transcription ofvapC20was induced by the addition of arabinose (0.2%) and total RNA was extracted from samples collected at time points indicated (min). The RNA was separated on 4.5% denaturing polyacrylamide gel and blotted onto a membrane, which was hybridized with radiolabelled probes KW-23S-3, KW-23S-1-3, KW-23S-2-3, KW-23S-3-3 and KW-23S-4-3 (Supplementary Table S2) indicated by numbers 1–5, respectively. Arrow points to the low-molecular-weight product. (d) Mapping of the VapC20 cleavage site inE. coli23S rRNA by primer extension analysis. RNA isolated as incwas hybridized with radiolabelled probe KW-23S-3-3 followed by cDNA synthesis by reverse transcription. The products were separated on a 6% denaturing polyacrylamide together with a sequencing ladder. MG1655 was also treated with 50 μg ml−1Cm and included as a control. The position of the VapC20 cleavage site within the SRL loop is indicated in the sequence with an arrow. Figure 2: VapC20 cleaves the SRL loop of 23S rRNA. ( a ) Analysis of total RNA from E. coli . MG1655/pKW82 (P BAD :: vapC MYSH ; left panel) and MG1655/pKW332549c (P BAD ::SD op :: vapC20 ; right panel) were grown exponentially in LB medium and transcription induced at time zero by the addition of arabinose (0.2%). Cell samples were collected at the time points indicated (min). Total RNA extracted from the samples were separated on a 4.5% denaturing polyacrylamide gel and visualized by ethidium bromide staining. M denotes an RNA size marker. VapC cleavage products are indicated with arrows. ( b ) The position of the probes used in c are indicated in the secondary structure of domain VI of 23S rRNA. The universally conserved nucleotides in the SRL loop of Helix 95 are indicated in green and the VapC20 cleavage site by an arrow. ( c ) Mapping of the cleavage site by northern blot analysis. Cells of MG1655/ pKW332549c (P BAD ::SD op :: vapC20 ) were grown exponentially in LB medium. At time zero, transcription of vapC20 was induced by the addition of arabinose (0.2%) and total RNA was extracted from samples collected at time points indicated (min). The RNA was separated on 4.5% denaturing polyacrylamide gel and blotted onto a membrane, which was hybridized with radiolabelled probes KW-23S-3, KW-23S-1-3, KW-23S-2-3, KW-23S-3-3 and KW-23S-4-3 ( Supplementary Table S2 ) indicated by numbers 1–5, respectively. Arrow points to the low-molecular-weight product. ( d ) Mapping of the VapC20 cleavage site in E. coli 23S rRNA by primer extension analysis. RNA isolated as in c was hybridized with radiolabelled probe KW-23S-3-3 followed by cDNA synthesis by reverse transcription. The products were separated on a 6% denaturing polyacrylamide together with a sequencing ladder. MG1655 was also treated with 50 μg ml −1 Cm and included as a control. The position of the VapC20 cleavage site within the SRL loop is indicated in the sequence with an arrow. Full size image VapC20 cleaves in the SRL loop To approach the cleavage position of VapC20 within 23S rRNA, we use northern blotting analysis by probing for a wide range of sites within domain VI of 23S rRNA ( Fig. 2b,c ). Probes 1 (probing 23S residues 2,870–2,889), 2 (residues 2,806–2,825), 3 (residues 2,722–2,742) and 4 (residues 2,674–2,692) all detect the low-molecular-weight cleavage band, whereas probe 5 (residues 2,621–2,640) does not, indicating that cleavage occur in region 2,640–2,674 containing 23S helix 95 and the universally conserved SRL loop. Finally, we use primer extension analysis to map the exact position of the cleavage site to between residues G2661 and A2662 in the SRL loop ( Fig. 2d ). Consistent with the northern blotting analysis, no cleavage is observed when cells are treated with Cm. VapC20 cleaves 23S rRNA of M. smegmatis at the exact same position (see Supplementary Fig. S3C ). To obtain purified, active VapC20, we purify a His-TEV-FLAG-tagged version of VapC20 (VapC20-HTF) from M. smegmatis and analyse the cleavage activity on an in vitro -transcribed 34 nucleotide SRL substrate (see Supplementary Fig. S4A ). No cleavage by VapC20 is observed even after extended incubation times. Next, we analyse VapC20 cleavage activity by northern blot analysis of purified total RNA using a probe specific for 23S rRNA ( Fig. 3a , lanes 1 and 2). Again, no band corresponding to cleavage within the SRL loop is observed (compare lanes 2 and 6 of Fig. 3a ). Weak unspecific cleavages are observed, indicating that the purified enzyme has ribonuclease activity. Finally, we analyse VapC20 cleavage activity using purified, intact ribosomes ( Fig. 3a lanes 3 and 4). Indeed, efficient site-specific cleavage of 23S rRNA is observed (compare lanes 4 and 6, see also Supplementary Fig. S4B for a time course of the cleavage reaction). Furthermore, treatment with a chelating agent (EDTA) abolishes in vitro cleavage by VapC20, consistent with Mg 2+ -dependent cleavage activity ( Fig. 3a , lane 5). Finally, the in vitro cleavage of VapC20 is mapped to occur between G2661 and A2662, identical to the result we observe in the in-vivo reaction ( Fig. 3b ). 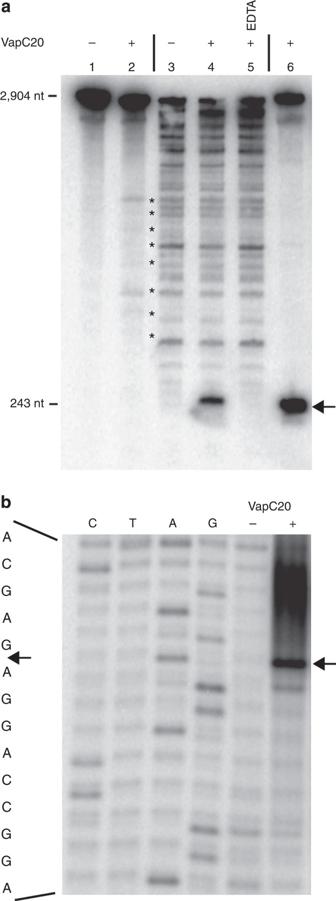Figure 3: VapC20 cleaves 23 rRNA of purified ribosomes. (a) Northern blot analysis ofin vitro-cleavedE. colitotal RNA and purified ribosomes. PurifiedE. colitotal RNA (lanes 1 and 2) or ribosomes (lanes 3–5) were incubated with or without purified VapC20-HTF (indicated by plus or minus) in cleavage buffer. EDTA was included in lane 5 as a control for the requirement of Mg2+in the reaction. Lane 6 shows total RNA purified fromE. colicells expressing VapC20 for 40 min. After incubation of the reactions in lane 1–5 for 10 min at 37 °C, VapC20 was inactivated by phenol/chloroform extraction and 1 μg of extracted RNA was separated on a 4.5% denaturing acrylamide gel. The RNA was subsequently blotted onto a membrane and 23S rRNA visualized by hybridization with32P-labelled KW-23S-3 probe. The cleavage products are indicated with an arrow; unspecific cleavages are indicated with asterisks. (b) Mapping of the VapC20in vitrocleavage site by primer extension analysis. Purified ribosomes (2 pmol) were incubated with or without 2 μg VapC20-HTF as ina. One microgram of extracted RNA was hybridized to32P-labelled probe KW-23S-3-3 followed by cDNA synthesis by reverse transcription. The cDNA products and a sequencing ladder were separated on a 10% denaturing polyacrylamide gel and visualized by phosphorimaging. The position of the cleavage site is indicated with arrows. Figure 3: VapC20 cleaves 23 rRNA of purified ribosomes. ( a ) Northern blot analysis of in vitro -cleaved E. coli total RNA and purified ribosomes. Purified E. coli total RNA (lanes 1 and 2) or ribosomes (lanes 3–5) were incubated with or without purified VapC20-HTF (indicated by plus or minus) in cleavage buffer. EDTA was included in lane 5 as a control for the requirement of Mg 2+ in the reaction. Lane 6 shows total RNA purified from E. coli cells expressing VapC20 for 40 min. After incubation of the reactions in lane 1–5 for 10 min at 37 °C, VapC20 was inactivated by phenol/chloroform extraction and 1 μg of extracted RNA was separated on a 4.5% denaturing acrylamide gel. The RNA was subsequently blotted onto a membrane and 23S rRNA visualized by hybridization with 32 P-labelled KW-23S-3 probe. The cleavage products are indicated with an arrow; unspecific cleavages are indicated with asterisks. ( b ) Mapping of the VapC20 in vitro cleavage site by primer extension analysis. Purified ribosomes (2 pmol) were incubated with or without 2 μg VapC20-HTF as in a . One microgram of extracted RNA was hybridized to 32 P-labelled probe KW-23S-3-3 followed by cDNA synthesis by reverse transcription. The cDNA products and a sequencing ladder were separated on a 10% denaturing polyacrylamide gel and visualized by phosphorimaging. The position of the cleavage site is indicated with arrows. Full size image VapC20 recognizes nucleotides flanking the cleavage site We developed a strategy to rapidly identify the VapC20 recognition elements in 23S rRNA in vivo . E. coli has seven operons encoding ribosomal RNAs; thus, the cleavage band generated by VapC20 in vivo ( Fig. 2 ) and in vitro ( Fig. 3 ) therefore consists of a mixture of cleavage products originating from several different 23S rRNAs. To obtain a uniform VapC20 substrate and to avoid potential toxicity, we therefore constructed a plasmid-based, conditional expression system that allows us to analyse VapC20 cleavage of 23S rRNA-derived fragments corresponding to a specific rrn operon ( rrlB ; Fig. 4a and Supplementary Fig. S5A ). To confirm the validity of the approach, we first analyse the full-length rrlB -encoded 23S rRNA, which indeed is cleaved in the SRL loop by VapC20 in vivo ( Fig. 4c , left panel). However, reducing the construct to an RNA substrate consisting of the SRL loop or an extended version of it, in both cases prevent cleavage by VapC20 (see Supplementary Fig. S5B ). 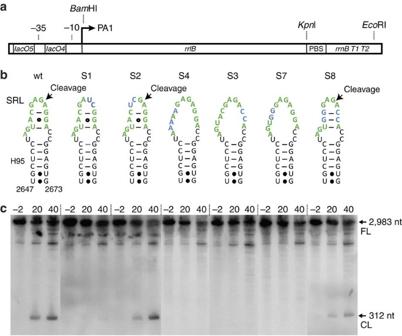Figure 4: VapC20 recognizes both primary and secondary structures of the SRL stem loop. (a) Schematic diagram showing the genetic setup of therrlB23S rRNA expression vector, including the positions of the IPTG-inducible PA1/O4/O5promoter, therrlBgene, the primer binding site (PBS) and therrnBT1T2 transcriptional terminator. (b) Primary and secondary structures of the SRL loop, stem and Helix 95 of 23S rRNA encoded by theE. coli rrlBgene. The universally conserved SRL stem loop bases are shown in green, base substitutions are in blue. (c) Northern blotting analysis onrrlBandrrlBtranscripts carrying the substitutions shown inb. We used a BW25113Δrnrstrain that lacks RNase R, as the rRNA fragment was more readily detected in this strain. Cells of BW25113Δrnrcontaining pKW332549c and either of therrlBconstructs pKW22PLT7AA (wtSRL), pKW22PLT7AAM1 (S1), pKW22PLT7AAM2 (S2), pKW22PLT7AAM3 (S3), pKW22PLT7AAM4 (S4), pKW22PLT7AAM7 (S7) or pKW22PLT7AAM8 (S8) were grown exponentially in LB medium at 37 °C. Twenty minutes before time zero (OD450~0.15), transcription ofrrlBwas induced by the addition of 2 mM IPTG. At time zero,vapC20was induced (0.2% arabinose) and samples taken at the time points indicated (min). Total RNA was extracted and the RNA separated on a 4.5% denaturing polyacrylamide gel. The RNA was subsequently blotted onto a membrane that was hybridized with32P-labelled KW-loop probe oligo. FL: 23S rRNA full-length transcript; CL: cleavage product of 23S rRNA. Figure 4: VapC20 recognizes both primary and secondary structures of the SRL stem loop. ( a ) Schematic diagram showing the genetic setup of the rrlB 23S rRNA expression vector, including the positions of the IPTG-inducible P A1/O4/O5 promoter, the rrlB gene, the primer binding site (PBS) and the rrnB T1T2 transcriptional terminator. ( b ) Primary and secondary structures of the SRL loop, stem and Helix 95 of 23S rRNA encoded by the E. coli rrlB gene. The universally conserved SRL stem loop bases are shown in green, base substitutions are in blue. ( c ) Northern blotting analysis on rrlB and rrlB transcripts carrying the substitutions shown in b . We used a BW25113 Δrnr strain that lacks RNase R, as the rRNA fragment was more readily detected in this strain. Cells of BW25113 Δrnr containing pKW332549c and either of the rrlB constructs pKW22PLT7AA ( wt SRL), pKW22PLT7AAM1 (S1), pKW22PLT7AAM2 (S2), pKW22PLT7AAM3 (S3), pKW22PLT7AAM4 (S4), pKW22PLT7AAM7 (S7) or pKW22PLT7AAM8 (S8) were grown exponentially in LB medium at 37 °C. Twenty minutes before time zero (OD 450 ~0.15), transcription of rrlB was induced by the addition of 2 mM IPTG. At time zero, vapC20 was induced (0.2% arabinose) and samples taken at the time points indicated (min). Total RNA was extracted and the RNA separated on a 4.5% denaturing polyacrylamide gel. The RNA was subsequently blotted onto a membrane that was hybridized with 32 P-labelled KW-loop probe oligo. FL: 23S rRNA full-length transcript; CL: cleavage product of 23S rRNA. Full size image Because of the site-specific primer binding site just downstream of the full-length rrlB gene ( Fig. 4a ), our construct allows us to introduce and detect effects of mutational changes in and around the SRL loop. First, we changed the two nucleotides on either side of the VapC cleavage site in the SRL loop. As seen from Fig. 4c , substitutions G2661U and A2662C (mutant S1 in Fig. 4b ) abolish VapC20 cleavage. In contrast, nearby substitutions in the SRL loop (G2659U and A2660C; S2) does not affect cleavage substantially ( Fig. 4c ). These results show that VapC20 recognizes the identity of the nucleotides flanking the cleavage site, whereas other nucleotides in the loop were not distinguished. VapC recognizes the structure of the SRL stem The SRL stem is an extension of 23S rRNA helix 95 consisting of three base pairs and two canonical C–G and A–U pairs flanking a central purine–purine mismatch (A·G) ( Fig. 4b ). To address the importance of the SRL stem in VapC20 recognition and cleavage, we introduced the substitutions G2655A, U2656A and C2658A located on the 5′-side of the SRL stem that destroy the secondary RNA structure but do not affect the sequence of the VapC20 cleavage site as shown above to be important (S4 in Fig. 4b ). Interestingly, this modification of the 23S rRNA abolishes VapC20 cleavage of the SRL loop, suggesting that the SRL stem structure is critical for VapC recognition and cleavage ( Fig. 4c ). To address whether the specific bases of the stem were important for recognition (provided the structure is present), we opened either side of the top of the SRL stem by changing two nucleotides (structures S3 and S7 in Fig. 4b ) and finally regenerated the secondary structure by combining the base changes of S3 and S7 into one construct (resulting in S8). In this experiment, both substitutions destroying the RNA secondary structure abolish VapC20 cleavage. In contrast, regeneration of the SRL stem restores significant cleavage (S8 in Fig. 4c ). This stem is different from that of the native SRL loop, perhaps explaining the slightly lower cleavage efficiency observed on this substrate. In conclusion, we have shown that the secondary structure rather than the sequence of the SRL stem structure is important for the recognition and cleavage by VapC20. Finally, given that we observe no cleavage of a simple construct containing only the SRL stem structure, we wanted to address whether tertiary interactions within the 23S rRNA are important for VapC recognition and cleavage. Within the 50S subunit, A2662 and G2663 (and partially C2658) of the SRL loop make direct contacts to A2531 and G2532 of helix 91 in domain V, thus potentially influencing VapC recognition (see Supplementary Fig. S5C ). Interestingly, however, the substitutions A2531C and G2532U that change the tertiary interactions with the SRL loop only weakly affect cleavage (see Supplementary Fig. S5D ). Therefore, it is likely to be that these tertiary interactions are of minor importance for VapC20 recognition of 23S rRNA. The work presented here establishes that VapC20 of M. tuberculosis is an endoribonuclease that cleaves between nucleotides G2661 and A2662 in helix 95 of 23S rRNA ( Fig. 2 ). These nucleotides form part of the longest universally conserved rRNA sequence known, the SRL loop. G2661 and A2662 are essential to the function of the SRL loop and were recently implicated in EF–Tu- and EF–G-mediated GTP hydrolysis [26] , [27] . During translation elongation, the SRL loop is also required for anchoring of EF–G to the ribosome during translocation [28] . Taken together, it is not surprising that cleavage of the SRL loop causes translational arrest and readily explains that VapC20 is a potent inhibitor of global translation ( Fig. 1 ). We find that VapC20 recognizes the nucleotides that flank the cleavage site but not other residues in the SRL loop region ( Fig. 4c ). Moreover, an intact secondary structure of the SRL stem is required for cleavage, whereas the exact sequence is not ( Figs 3a and 4c ). Perhaps surprisingly, VapC20 does not cleave the isolated SRL fragments of 23S rRNA used in this paper neither in vitro nor in vivo , suggesting that additional regions of the 50S subunit or the ribosome are recognized or the presence of ribosomal proteins are needed for VapC20 to bind. Analysis of the crystal structure of the intact Thermus thermophilus 70S ( Fig. 5a ) shows that helix 95 and the SRL loop are exposed on the surface of the ribosome and therefore would be readily accessible [29] . In addition, the cleavage site within the SRL loop (marked with dark red in Fig. 5a ) is facing towards the outside and a relatively large cavity between the ribosomal subunits. This suggests that VapC20 has direct access to the ribosomal cleavage site. 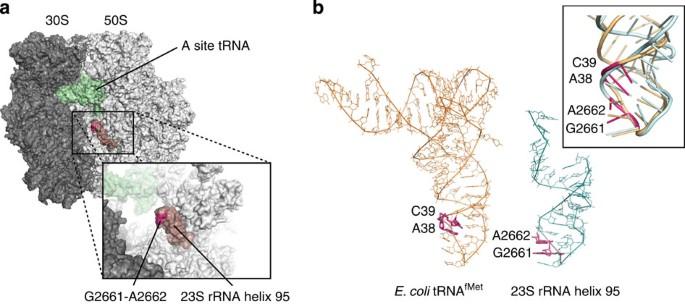Figure 5: Visualization of the VapC20 target site inside 23S ribosomal RNA. (a) Structural overview of the bacterial ribosome (T. thermophilus, PDB IDs 3ZN7 and 3ZN9)29with the 50S subunit in light grey and the 30S subunit in dark grey. The APE tRNAs are shown in green with the A site tRNA in front. Helix 95 of 23S rRNA is coloured dark pale red with the cleavage site in bright magenta. The inset shows a close-up of helix 95 highlighting the nearby cavity between the two subunits. (b) Side-by-side comparison of the RNA targets of VapC from enteric bacteria, tRNAfMet(exemplified by theE. colitRNAfMet, PDB ID 3CW5)30, shown to the left in gold and that of VapC20, 23S helix 95 or the SRL (T. thermophilus23S, PDB ID 3ZN9)29, right, blue. In both cases, the two nucleotides flanking the cleavage site are highlighted with magenta sticks and labelled. The inset shows a structural superpositioning of the two RNA targets using the same colouring scheme. Figure 5: Visualization of the VapC20 target site inside 23S ribosomal RNA. ( a ) Structural overview of the bacterial ribosome ( T. thermophilus , PDB IDs 3ZN7 and 3ZN9) [29] with the 50S subunit in light grey and the 30S subunit in dark grey. The APE tRNAs are shown in green with the A site tRNA in front. Helix 95 of 23S rRNA is coloured dark pale red with the cleavage site in bright magenta. The inset shows a close-up of helix 95 highlighting the nearby cavity between the two subunits. ( b ) Side-by-side comparison of the RNA targets of VapC from enteric bacteria, tRNA fMet (exemplified by the E. coli tRNA fMet , PDB ID 3CW5) [30] , shown to the left in gold and that of VapC20, 23S helix 95 or the SRL ( T. thermophilus 23S, PDB ID 3ZN9) [29] , right, blue. In both cases, the two nucleotides flanking the cleavage site are highlighted with magenta sticks and labelled. The inset shows a structural superpositioning of the two RNA targets using the same colouring scheme. Full size image Given that enteric VapCs and VapC20 belong to the same subgroup of ribonucleases (the PIN domain proteins) that have similar tertiary folds, it is likely to be that they approach, recognize and cleave their RNA targets by similar mechanisms. However, such speculation leaves open the question of how they are able to specifically recognize very different targets. In the general view, both VapC nucleases recognize and cleave RNA stem loop structures, namely the 23S SRL loop and the anticodon loop of tRNA fMet . Investigation of the two stem loop structures ( Fig. 5b ) shows that they share many structural features ( Fig. 5b inset) and, furthermore, that the observed cleavage site is on the same side of the stem structure with respect to the terminal tetraloop [29] , [30] . However, there are also clear differences between them: although VapC20 cleaves in the tetraloop region of the SRL stem loop, VapCs from enteric bacteria cleave further up the A-form tRNA anticodon stem. In addition, the SRL loop shows significant deviations from standard A-form RNA in the stem. Together, this suggests that subtle structural differences are important reasons as to why two nucleases, which are most likely to be structurally very similar, are able to specifically cleave very different cellular target RNAs. Although both VapC20 and VapCs from enteric bacteria are highly specific ribonucleases with only one distinct cellular target each (ref. 15 and this work), other prokaryotic VapCs exhibit nonspecific RNase activity in vitro [9] , [31] , [32] , [33] , [34] or cleave degenerated recognition motifs in synthetic RNAs [35] , [36] . Further, in one case (VapC4 of M. tuberculosis ), the presumed PIN-domain ribonuclease binds in vitro to RNAs containing the motif ACGC and is suggested to inhibit translation by stoichiometric binding to mRNAs containing such recognition motifs [20] . Interestingly, when we use Mn 2+ instead of Mg 2+ in in vitro reactions with enteric VapCs, the ribonucleases degraded RNA nonspecifically [19] . In addition, when VapC20 is incubated with purified total RNA (primarily rRNA) weak unspecific cleavage is observed ( Fig. 3a , lane 2). Thus, the in vitro specificities of the site-specific VapC RNases are highly influenced by the assay conditions and it cannot be excluded that some of the VapCs described to be nonspecific RNases actually may be more specific when tested under different conditions. Fungal ribotoxins, such as α-Sarcin and several others, cleave the SRL loop at the exact same position as VapC20, that is, between nucleotides G2661 and A2662 (ref. 37 ). PIN domains are divalent metal ion-dependent RNases with active sites similar to RNase H that generate cleavage products with 3′-hydroxyl groups [38] . In contrast, Sarcin-like ribotoxins belong to the RNase T1 class of ribonucleases that generate cleavage products with 3′-cyclic phosphate groups [37] . Thus, even though VapC20 and α-Sarcin are structurally unrelated and cleave RNA by different enzymatic mechanisms, they represent an unusual example of convergent evolution at the functional level. In the following, we discuss two possible biological functions of vapBC20 . First, there is experimental evidence supporting that some type II TAs and, in particular, type III TAs function as defence systems against bacteriophages [39] , [40] . In this scenario, entry of a bacteriophage into a host bacterium activates a toxin by stimulating the degradation of the cognate antitoxin. In turn, the activated toxin inhibits translation and thereby aborts the formation of novel virus progeny. Second, vapBC20 may function in persistence and multidrug tolerance, as in the case of TAs of E. coli . Similar to E. coli , many TAs of M. tuberculosis were induced in persister cells [10] , [41] . Given that VapC20 inhibits translation, it is possible that vapBC20 functions in persistence. Consistently, a significant proportion of VapC20-inhibited cells could be resuscitated upon induction of vapB20 ( Fig. 1d ). It is now important to unravel the biological functions of TA modules not only in M. tuberculosis but also in other pathogenic bacteria. The work presented here represents an important step in this challenging and exciting endeavour. Strains and growth conditions E. coli K-12 and M. smegmatis mc 2 155 were grown in Lysogeny broth (LB medium) at 37 °C. For M. smegmatis , LB medium was supplemented with 0.05% Tween-80 (called LBT medium). In some experiments, E. coli was grown in M9 minimal medium with appropriate amino acids and 0.5% glycerol as the carbon source. When appropriate, 50 μg ml −1 Cm, 30 μg ml −1 ampicillin, 50 μg ml −1 kanamycin or 100 μg ml −1 hygromycin B were added to growth media to maintain plasmids. When stated, 2 mM IPTG, 0.2% arabinose or 20 ng ml −1 tetracycline was added to growth medium or solid media to induce transcription of either vapC20 or vapB20 . Strains are listed in Supplementary Table S2 . Plasmids Plasmids constructed are described in Supplementary Methods and also listed in Supplementary Table S1 . Oligonucleotides are listed in Supplementary Table S2 . Viable counts Overnight cultures of MG1655 containing pBAD33, pKW332549c, pKW222550cop or pKW222550copLL were diluted in LB medium to OD 450 ≈0.005 and grown under aeration at 37 °C. At OD 450 ≈0.5, the cultures were diluted ten times and growth continued. When the cultures reached OD 450 ≈0.4, vapC20 transcription was induced by addition of arabinose (0.2%). Samples were diluted and plated on solid medium containing appropriate antibiotics and 0.2% glucose. When indicated, plates were supplemented with IPTG (2 mM). The colonies were counted and plotted as CFU ml −1 . Pulse-chase experiments MG1655/pKW332549c was grown exponentially in synthetic M9 medium containing all amino acids, except methionine and 0.5% glycerol as the carbon source. At OD 450 =0.3–0.4, the cultures were induced with 0.2% arabinose. Samples (0.5 ml) were pulsed for 1 min with radiolabelled 35 S-methionine (10 μCi), 3H-methyl-thymidine (2 μCi) or 3 H-uridine (2 μCi) with 100-fold excess of unlabelled methionine, thymidine or uridine as carriers, at 37 °C. Subsequently, samples were chased by addition of 5 × 10 6 -fold excess of unlabelled methionine, thymidine or uridine for 5 min at 37 °C. Protein, RNA and DNA were precipitated by addition of ice-cold trichloroacetic acid to a final concentration of 20% and were collected by centrifugation for 30 min at 4 °C. The precipitate was then washed twice in ice-cold 100% ethanol and resuspend in 200 μl 1% SDS. The incorporation of radioisotopes was then measured by liquid scintillation counting. Extraction of total RNA from E. coli Total RNA was prepared using hot phenol/chloroform extractions. Cell samples were resuspend in 200 μl ice-cold solution I (0.3 M sucrose, 0.01 M Na-acetate, pH 4.5) and rapidly mixed with 200 μl solution II (2% SDS, 0.01 M Na-acetate, pH 4.5) and 400 μl phenol, pH 4.5 (Sigma). Samples were then vortexed for 1 min and incubated at 65 °C for 3 min. The solution was then submerged in liquid nitrogen and centrifuged for 5 min at room temperature. After centrifugation, the top phase was extracted with 400 μl phenol and the vortexing, heating, freezing and centrifugation step was repeated. The top phase was then mixed with 400 μl chloroform and vortexed for 1 min, followed by centrifugation for 5 min at room temperature. The RNA was then precipitated from the top phase by mixing it with 100 μl 1 M Na-acetate, pH 4.5, and 1 ml ice-cold ethanol, and leaving the solution at −20 °C for a minimum of 30 min. The RNA was finally collected by centrifugation at maximum speed for 30 min at 4 °C. The RNA pellet was briefly washed in ice-cold 70% ethanol before being dried at room temperature and resuspend in nuclease-free water. Extraction of total RNA from M. smegmatis Total RNA was extracted using FastRNA Blue Kit (MP Biomedicals) followed by phenol/chloroform extractions. Initial RNA extraction was performed according to manufactures instructions. Cell samples were dissolved in 1 ml RNA pro solution and transferred to a 2-ml tube containing Lysing matrix B. The cells were then lysed by processing the tube in Precellys 24-cell homogenizer (Bertin Technologies) for two cycles of 40 s at 6,500 r.p.m., separated by a 1 min rest at 4 °C. The solution was then centrifuged for 5 min at 4 °C. The supernatant was carefully transferred to a new tube containing 300 μl chloroform, vortexed and incubated for 5 min on ice before centrifugation at for 5 min at 4 °C. The top phase was then mixed with 600 μl ethanol and incubated for at least 30 min at −20 °C. The RNA precipitate was then collecetd by centrifugation for 20 min at 4 °C. The pellet was resuspended in 300 μl 0.1 M Na-acetate, pH 4.5, followed by two extractions: once with 400 μl phenol and once with 400 μl chloroform. The top phase was then mixed with 100 μl 1 M Na-acetate, pH 4.5, and 1 ml ice-cold ethanol, and then left to precipitate at −20 °C for least 30 min. Finally, the RNA was collected, washed in 70% ice-cold ethanol, dried and resuspend in nuclease-free water. Northern blotting analysis For detection of 16S and 23S rRNAs, 2.5 or 15 μg of total RNA was separated on a 4.5% denaturing polyacrylamide gel in 1 × Tris-borate-EDTA buffer. The RNA was then transferred to a zeta-probe membrane (Bio-Rad) by electroblotting in 1 × Tris-borate-EDTA buffer. The membrane was subsequently hybridized overnight at 42 °C with appropriate radiolabelled oligonucleotide probe in 1 × PerfectHyb Plus hybridization buffer (Sigma). The oligonucleotides (~14 pmol) were 5′-end labelled using T4 polynucleotide kinase (NEB) and 10 μCi of [γ 32 P]-ATP, and added to the membrane after prehybridization for 5 min. For the detection of E. coli K-12 16S and 23S rRNA, oligonucleotides KW-16S-3, KW-23S-3, KW23S-1-3, KW-23S-2-3, KW-23S-3-3 and KW-23S-4-3 were used. For the detection 23S rRNA of M. smegmatis mc 2 155, the KW-MS-23S-II oligonucleotide was used. For the detection of 23S rRNA transcribed from plasmids, pKW22PLT1, pKW22PLT4, pKW22PLT6, pKW22PLT7AA, pKW22PLT7AAM1, pKW22PLT7AAM2, pKW22PLT7AAM3, pKW22PLT7AAM4, pKW22PLT7AAM5, pKW22PLT7AAM7 and pKW22PLT7AAM8 oligonucleotide KW-loop probe were used. After hybridization, the blot was washed two to three times in 2 × saline-sodium-citrate buffer with 0.1% SDS at room temperature. 32 P was detected by phosphorimaging. Detection of tRNA by northern blotting Five micrograms of total RNA was prepared from E. coli cells and separated on an 8% denaturing polyacrylamide gel in 0.1 M Na-acetate, pH 5. The RNA was transferred to a Hybond-N membrane (GE Healthcare) by electroblotting in 40 mM Tris-acetate, pH 8.2, and 2 mM EDTA. The membrane was then hybridized with appropriate DNA oligonucleotides and tRNA detected as described for 16S and 23S rRNA. The following DNA oligonucleotides were used: KW-tRNAfMet, KW-tRNA1Thr, KW-tRNAHis, KW-tRNAPhe, KW-tRNA2Arg, KW-tRNATyr and KW-tRNAVal. Primer extension analysis Oligonucleotides KW-23S-3-3 and KW-MS23S-3-II were used to map the VapC20 cleavage site in 23S rRNA of E. coli K-12 and M. smegmatis mc 2 155, respectively. Four picomoles of primer was labelled with 30 μCi of [γ 32 P]-ATP using T4 polynucleotide kinase and subsequently cleaned/desalted using Illustra microspin G-25 columns (GE Healthcare). One microgram of total RNA was hybridized with 0.2 pmol of labelled oligonucleotide in a total volume of 6 μl by incubation at 80 °C for 10 min and leaving the sample on ice for 5 min. The oligonucleotides/RNA hybrids were then extended using SuperScript II reverse transcriptase (Invitrogen). To each hybridization, 2 μl 5 × FirstStrand buffer, 1 μl 0.1 M dithiothreitol (DTT) and 1 μl 10 mM dNTP were added and the reaction was placed at 45 °C. After 5 min of incubation, 1 μl of Superscript II reverse transcriptase (diluted 1:10) was added and the reaction was incubated for 1 h at 45 °C. The reaction was stopped by the addition of formamide loading buffer and the complementary DNA separated on a 6% denaturing polyacrylamide gel. The site of cleavage was determined from a dideoxy sequence ladder generated from PCR products using primers KW-23S-3-3 and KW-23S-PXT for E. coli K-12 23S rRNA and KW-MS-23S-3-II and KW-MS-23S-PXT for M. smegmatis mc 2 155 23S rRNA. The sequence ladder and cDNA were detected by phosphorimaging. Purification of VapC20-HTF Native VapC20-HTF was purified from Mycobacterium smegmatis using histidine affinity chromatography. Strain Mc 2 155/pMIND-GTG-Rv2549c-HTF was grown exponentially in 1 litre LBT at 37 °C with shaking. At OD 600 =0.4, the culture was induced with 20 ng ml −1 tetracycline for 1 h before cells were pelletted by centrifugation. The cells were then washed in ice-cold PBS containing 0.1% Tween-80 and lysed in 1 ml (v/w) lysis buffer (50 mM NaH 2 PO 4 , pH 8, 300 mM NaCl, 10 mM imidazole, 0.1% NP-40, 5 mM β-mercaptoethanol) by bead beating (2 × 6,500 r.p.m. for 40 s, Precellys 24-cell homogenizer) using 0.5 ml 100 μM glass beads per 1.5 ml of cells. The lysate was cleared by centrifugation at 14,000 r.p.m. for 20 min and incubated overnight at 4 °C with 0.5 ml Ni-NTA resin (Qiagen). The resin was then loaded onto a gravity-flow column and washed with 20 column volume of wash buffer (50 mM NaH 2 PO 4 , pH 8, 300 mM NaCl, 20 mM imidazole, 0.1% NP-40, 5 mM β-mercaptoethanol). VapC20-HTF was then eluted by a 2-ml stepwise increase in imidazole concentration. Western blot analysis confirmed protein to be eluting between 80 and 160 mM imidazole. Fractions containing VapC20-HTF were pooled and dialysed for 6 h against PBS containing 1 mM DTT and overnight against PBS containing 20% glycerol and 1 mM DTT at 4 °C. In vitro cleavage assay Purified total RNA (3 μg) or intact ribosomes (2 pmol) from E. coli K-12 were incubated with 2 μg VapC20-HTF for 2–10 min in cleavage buffer (10 mM HEPES, pH 7.5, 15 mM KCl, 10 mM MgCl 2 , 10% glycerol, 1 mM DTT) at 37 °C. VapC20-HTF was inactivated and by phenol/chloroform extractions and cleaved RNA precipitated with 100 μl Na-acetate, pH 4.5, 20 μg glycogen and three volumes of ice-cold ethanol for 30 min at −80 °C. The RNA was resuspended in nuclease-free water and 1 μg of RNA analysed by northern blotting using probe KW-23S-3 or primer extension analysis using probe KW-23S-3-3. How to cite this article: Winther, K. S. et al. VapC20 of Mycobacterium tuberculosis cleaves the Sarcin–Ricin loop of 23S rRNA. Nat. Commun. 4:2796 doi: 10.1038/ncomms3796 (2013).